Unravelling the mechanism of non-ribosomal peptide synthesis by cyclodipeptide synthases Cyclodipeptide synthases form cyclodipeptides from two aminoacyl transfer RNAs. They use a ping-pong mechanism that begins with transfer of the aminoacyl moiety of the first aminoacyl tRNA onto a conserved serine, yielding an aminoacyl enzyme. Combining X-ray crystallography, site-directed mutagenesis and affinity labelling of the cyclodipeptide synthase AlbC, we demonstrate that the covalent intermediate reacts with the aminoacyl moiety of the second aminoacyl tRNA, forming a dipeptidyl enzyme, and identify the aminoacyl-binding sites of the aminoacyl tRNAs. Cyclodipeptide synthases (CDPSs) are a novel family of enzymes that hijack aminoacyl tRNAs (aa-tRNAs) from their canonical function in ribosomal protein synthesis to produce various cyclodipeptides, which are precursors of many secondary metabolites with diverse biological activities [1] , [2] , [3] . They employ a ping-pong-type catalytic mechanism beginning with the binding of a first aa-tRNA and the transfer of its aminoacyl moiety onto a conserved serine leading to the formation of an aminoacyl enzyme intermediate [4] , [5] , [6] , [7] . The subsequent steps of the catalytic mechanism have not yet been elucidated. It has been proposed that the aminoacyl enzyme reacts with the aminoacyl moiety of a second aa-tRNA to form either a dipeptidyl enzyme [6] or a dipeptidyl tRNA intermediate [5] , which undergoes intramolecular cyclization to generate the final cyclodipeptide product ( Fig. 1 ). Neither of these two putative intermediates has ever been detected directly. 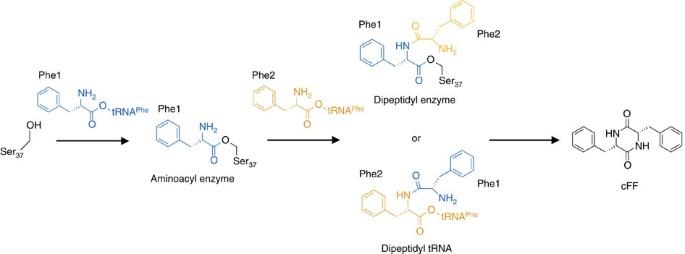Figure 1: Formation of cyclo(L-Phe-L-Phe) catalysed by the CDPS AlbC. The existence of the phenylalanyl AlbC intermediate was demonstrated previously4, but the nature of the dipeptidyl intermediate was unknown. Figure 1: Formation of cyclo( L -Phe- L -Phe) catalysed by the CDPS AlbC. The existence of the phenylalanyl AlbC intermediate was demonstrated previously [4] , but the nature of the dipeptidyl intermediate was unknown. Full size image The crystal structures of three CDPSs have been determined: AlbC from Streptomyces noursei , Rv2275 from Mycobacterium tuberculosis and YvmC from Bacillus licheniformis [4] , [5] , [6] . These enzymes possess a common architecture very similar to the catalytic domains of class-I aa-tRNA synthetases (aaRSs), especially class-Ic TyrRSs and TrpRSs. In particular, the aminoacyl moiety of the first aa-tRNA substrate of CDPS is thought to bind in a pocket [4] , [5] , [6] , [7] , structurally corresponding to the tyrosine-binding pocket in TyrRSs (PDB 1J1U [8] ). Accordingly, buffer components were identified within this pocket in several CDPS crystal structures [4] , [6] . However, no structure of a CDPS in complex with either a natural substrate or a ligand representative of a reaction intermediate has been obtained. Here we present the first crystal structure of a CDPS complexed with a reaction intermediate analogue. This structure, combined with site-directed mutagenesis and chemical biology experiments, reveals that the second reaction intermediate is a dipeptidyl enzyme. We map the aminoacyl-binding sites for each of the two aa-tRNA substrates. Finally, we identify the residue responsible for the intramolecular cyclization of the dipeptidyl intermediate and revisit the roles of the other active site residues. We reasoned that the identification of the second reaction intermediate would be facilitated by blocking the enzymatic reaction before dipeptide cyclization. To identify residues possibly involved in cyclization, we first determined the crystal structure of a complex mimicking a putative dipeptidyl AlbC intermediate. AlbC synthesizes cyclo( L -Phe- L -Leu) (cFL) and cyclo( L -Phe- L -Phe) (cFF) [2] , and its S37 residue is the target for phenylalanylation [4] ( Fig. 1 ). Therefore, if a dipeptidyl enzyme intermediate indeed occurs, it should be composed of a dipeptide covalently linked by its carboxylate terminus to the S37 hydroxyl. To obtain a structural analogue of L -Phe- L -Phe-AlbC, we used N -carbobenzyloxy- L -Phe-chloromethyl ketone (ZPCK) ( Fig. 2a ), a molecule close to the Phe-Phe dipeptide ( Fig. 1 ). We used the active AlbC variant S37C [4] as a target for ZPCK labelling, because the chloromethyl ketone in this analogue is able to react with thiol groups ( Fig. 2a ). As expected, trypsin digestion and peptide mass fingerprinting (PMF) showed that C37 was covalently modified after incubation of AlbC S37C with ZPCK ( Supplementary Fig. 1 ). 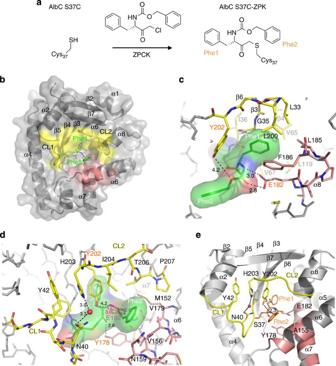Figure 2: Affinity labelling of AlbC and crystal structure of a complex mimicking the dipeptidyl enzyme intermediate. (a) The AlbC variant S37C was covalently modified withN-carbobenzyloxy-L-Phe-chloromethyl ketone (ZPCK). The labelled CDPS was named AlbC S37C-ZPK. (b) Cartoon representation of the structure of AlbC S37C-ZPK (PDB4Q24). Secondary structure elements are labelled. The protein is shown in grey as a semi-transparent molecular surface. Regions surrounding the ZPK adduct are coloured as follows: CL1 and CL2 (CL1: 33–43, CL2: 202–207), and the N terminus of β3,4,6 are in yellow. Parts of α6 (151–159) and α7 (172–182) are in pink. Phe1 is buried deep within its cavity, whereas Phe2 lies in a wide pocket. (c) Close-up view of the Phe1-binding site. The ZPK adduct is shown as green sticks within its molecular surface. Residues delineating the cavities are shown as sticks; catalytic residues are labelled in orange. Yellow is used for β-strands and pink for helix α8. Relevant interactions are indicated with a dashed line. (d) Close-up view of the Phe2-binding site. Yellow is used for CL1 and CL2, and pink for α6 and α7. Important residues are shown as sticks; catalytic residues are labelled in orange. This view highlights stacking interactions between Y42, H203 and Y202, and a water-mediated interaction between N40 and H203 that stabilize the positions of CL1 and CL2. Notably, a water molecule is present at the same position in the active site of Rv2275. Y178, E182 and Y202 are in close proximity to ZPK. Hydrogen bonds between Y178 and E182 are indicated with dashed lines. (e) Model of the diphenylalanyl enzyme. Position of the diphenylalanyl adduct was modelled according to the position of the ZPK adduct (Supplementary Fig. 6). The diphenylalanyl adduct was constructed with the REEL and eLBOW programmes from the Phenix suite28. Important regions involved in the binding of the dipeptide are in yellow and pink. The dipeptide intermediate is shown as orange sticks. Important residues are shown as sticks. According to this model, the oxygen group of Y202 is positioned 3.1 Å away from the NH2group of the dipeptide. All structural drawings were done with PYMOL (www.pymol.org). Figure 2: Affinity labelling of AlbC and crystal structure of a complex mimicking the dipeptidyl enzyme intermediate. ( a ) The AlbC variant S37C was covalently modified with N -carbobenzyloxy- L -Phe-chloromethyl ketone (ZPCK). The labelled CDPS was named AlbC S37C-ZPK. ( b ) Cartoon representation of the structure of AlbC S37C-ZPK (PDB 4Q24 ). Secondary structure elements are labelled. The protein is shown in grey as a semi-transparent molecular surface. Regions surrounding the ZPK adduct are coloured as follows: CL1 and CL2 (CL1: 33–43, CL2: 202–207), and the N terminus of β3,4,6 are in yellow. Parts of α6 (151–159) and α7 (172–182) are in pink. Phe1 is buried deep within its cavity, whereas Phe2 lies in a wide pocket. ( c ) Close-up view of the Phe1-binding site. The ZPK adduct is shown as green sticks within its molecular surface. Residues delineating the cavities are shown as sticks; catalytic residues are labelled in orange. Yellow is used for β-strands and pink for helix α8. Relevant interactions are indicated with a dashed line. ( d ) Close-up view of the Phe2-binding site. Yellow is used for CL1 and CL2, and pink for α6 and α7. Important residues are shown as sticks; catalytic residues are labelled in orange. This view highlights stacking interactions between Y42, H203 and Y202, and a water-mediated interaction between N40 and H203 that stabilize the positions of CL1 and CL2. Notably, a water molecule is present at the same position in the active site of Rv2275. Y178, E182 and Y202 are in close proximity to ZPK. Hydrogen bonds between Y178 and E182 are indicated with dashed lines. ( e ) Model of the diphenylalanyl enzyme. Position of the diphenylalanyl adduct was modelled according to the position of the ZPK adduct ( Supplementary Fig. 6 ). The diphenylalanyl adduct was constructed with the REEL and eLBOW programmes from the Phenix suite [28] . Important regions involved in the binding of the dipeptide are in yellow and pink. The dipeptide intermediate is shown as orange sticks. Important residues are shown as sticks. According to this model, the oxygen group of Y202 is positioned 3.1 Å away from the NH 2 group of the dipeptide. All structural drawings were done with PYMOL ( www.pymol.org ). Full size image We solved the structure of the modified AlbC S37C, named AlbC S37C-ZPK (ZPK corresponds to N -carbobenzyloxy- L -Phe-methyl ketone), by molecular replacement using the previously determined unmodified AlbC structure (PDB 3OQV ). The resulting electron density map showed a supplementary mass of electron density connected to C37, and some rearrangements in the structure of the enzyme. The supplementary density clearly corresponded to ZPK ( Supplementary Fig. 2 ). The structure was refined at 2.9 Å resolution after a few cycles of model fitting and energy minimization ( Table 1 ). The structural model consists of the entire AlbC S37C enzyme bound to ZPK ( Fig. 2b ), excluding residues 1–9 and residues 234–239 at the C-terminal extremity for which no electron density was visible. Overall, the AlbC S37C-ZPK structure is highly similar to the unmodified AlbC structure (root mean squared deviation=0.9 Å over 169 Cα, Supplementary Figs 3 and 4 ). However, the region linking the β6 and β7 strands, in the vicinity of the ZPCK binding site, is rearranged (residues 202–225). The 202–207 loop and α8 (residues 208–213) are pushed away from the active site cavity in the AlbC S37C-ZPK structure ( Fig. 2b and Supplementary Figs 3 and 4 ). In the structure of unmodified AlbC (PDB 3OQV ), Y202 and neighbouring residues are involved in crystal packing ( Supplementary Fig. 5 ). Therefore, the conformational difference of the 202–225 region between AlbC S37C-ZPK and unmodified AlbC cannot be attributed to modification by ZPK. Notably, the conformation of this region in AlbC S37C-ZPK appears close to that observed in Rv2275 and YvmC (PDB 2X9Q and 3OQJ , respectively; Supplementary Fig. 4 ). Table 1 Data collection and refinement statistics for AlbC S37C-ZPK structure determination. Full size table The aromatic ring (Phe1) of ZPK is buried deep within a hydrophobic pocket, corresponding to that occupied by cyclo-dithiothreitol in the AlbC structure [4] , or by the buffer components CHES or CAPSO in the structure of YvmC [6] . The cavity is delineated on one side by strands β3, β4 and β6, and on the other side by helix α8. In particular, there is a stacking interaction between F186 and the Phe1 ring ( Fig. 2c ). In the S37C-ZPK structure, the benzyl ring (Phe2) lies in a wider cavity delineated by two loops, hereafter named CL1 and CL2 (catalytic loop 1: residues 36–43; catalytic loop 2: residues 202–207), the C-terminal part of α6 (152–159) and the central part of α7 (175–183) ( Fig. 2d ). Stacking interactions involving Y42, H203 and Y202, and a water-mediated interaction between N40 and H203, stabilize the positions of the two catalytic loops. Notably, in AlbC S37C-ZPK the position of CL1 and CL2 places the side chain of Y202 in proximity to ZPK ( Fig. 2c,d ). We derived a model of the dipeptidyl enzyme from the AlbC S37C-ZPK structure ( Fig. 2e and Supplementary Fig. 6 ) and used it to identify residues possibly involved in dipeptide cyclization. The intramolecular cyclization of the dipeptide ester requires that the dipeptide be in a cis conformation to place the primary ammonium group in close proximity to the ester [9] , [10] . The conformation adopted by the dipeptide places the ammonium group of Phe2 near the ester carbonyl (2.3 Å), which is in line with this requirement ( Fig. 2e and Supplementary Fig. 6 ). This primary ammonium group should be deprotonated by a catalytic base to generate the nucleophile for attack at the activated ester. The conserved Y202 residue is a good candidate to fulfill this role, because its hydroxyl would be close to the ammonium group of Phe2 (3.1 Å) ( Fig. 2e and Supplementary Fig. 6 ). Such a role for a Y residue is unusual but has already been described [11] , [12] , [13] . In Rv2275 and YvmC, this residue was initially proposed to position and increase the nucleophilicity of the catalytic serine [5] , [6] . However, we showed previously that its substitution with a phenylalanine in AlbC did not affect the formation of the aminoacyl enzyme intermediate, demonstrating that Y202 is not responsible for the activation of the catalytic serine [4] . The Y202 hydroxyl is nevertheless essential, because the Y202F variant has 20-fold lower enzymatic activity than the wild-type enzyme, although its structural integrity is not affected ( Supplementary Table 1 and Supplementary Fig. 7 ). We hypothesized that the modification of Y202 to F may impair the cyclization process, allowing the trapping of the dipeptidyl enzyme if it indeed occurs. We incubated briefly the Y202F variant with two equivalents of Phe-tRNA Phe and immediately analysed the resulting species by liquid chromatography–mass spectrometry (LC–MS) or PMF. LC–MS analysis showed a mixture of three species, with masses consistent with the unmodified AlbC Y202F, a phenylalanyl enzyme and a diphenylalanyl enzyme ( Supplementary Fig. 8 ). Previous PMF analyses of trypsin-digested AlbC and of its Y202F variant gave two fragments containing the catalytic S37 (fragments [29–46] and [27–46]) [4] ( Supplementary Fig. 9 ). The PMF analysis of Y202F incubated with two equivalents of Phe-tRNA Phe gave the [27–46] fragment, low amounts of the [29–46] fragment and two additional fragments ( Fig. 3 ). The m/z of these two fragments were 2,310.17 and 2,457.2, and corresponded to the values expected for the addition of phenylalanyl and diphenylalanyl moieties on fragment [27–46], respectively. We sequenced unambiguously by both b - and y -series the fragment with an m/z of 2,457.2, which showed that it contained a diphenylalanyl adduct on S37. This experiment thus demonstrates the formation of the covalent dipeptidyl enzyme intermediate. Moreover, we did not observe the diphenylalanyl adduct with wild-type AlbC; therefore, we conclude that Y202 is involved in the cyclization process, probably by deprotonating the primary ammonium group. 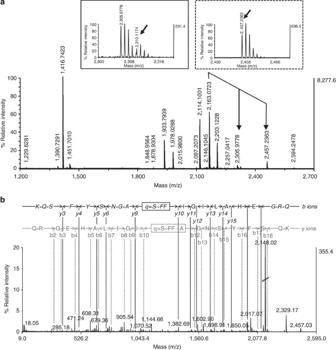Figure 3: Identification of the covalent dipeptidyl enzyme intermediate with the variant Y202F. (a) PMF analysis of trypsin-digested Y202F variant pre-incubated with two equivalents of Phe-tRNAPhefor 30 s. Arrows indicate the formation of two additional fragments that were not observed in the PMF analysis of the trypsin-digested Y202F variant not incubated with Phe-tRNAPhe(Supplementary Fig. 9): them/zat 2,310.12 (close-up view in solid box) corresponds to the potential phenylalanylated fragment [27–46] and them/zat 2,457.24 (close-up view in dashed box) corresponds to the diphenylalanylated fragment [27–46]. The non-modified [27–46] fragment was detected atm/z2,163.07. (b) PSD-MS/MS spectrum ofm/z2,457.24. Bothb- andy-ion series identify the amino acid sequence of the modified AlbC fragment [27–46] and identify the residue 37 as the diphenylalanylated residue. The main daughter-ion atm/z2,148.02 corresponds to the modified fragment [27–46] without its diphenylalanyl moiety. Note that the scale of the 2,148.02 peak differs from the others. Figure 3: Identification of the covalent dipeptidyl enzyme intermediate with the variant Y202F. ( a ) PMF analysis of trypsin-digested Y202F variant pre-incubated with two equivalents of Phe-tRNA Phe for 30 s. Arrows indicate the formation of two additional fragments that were not observed in the PMF analysis of the trypsin-digested Y202F variant not incubated with Phe-tRNA Phe ( Supplementary Fig. 9 ): the m/z at 2,310.12 (close-up view in solid box) corresponds to the potential phenylalanylated fragment [27–46] and the m/z at 2,457.24 (close-up view in dashed box) corresponds to the diphenylalanylated fragment [27–46]. The non-modified [27–46] fragment was detected at m/z 2,163.07. ( b ) PSD-MS/MS spectrum of m/z 2,457.24. Both b - and y -ion series identify the amino acid sequence of the modified AlbC fragment [27–46] and identify the residue 37 as the diphenylalanylated residue. The main daughter-ion at m/z 2,148.02 corresponds to the modified fragment [27–46] without its diphenylalanyl moiety. Note that the scale of the 2,148.02 peak differs from the others. Full size image The AlbC S37C-ZPK structure allowed us to revisit the role of other active site residues and propose the following catalytic mechanism ( Fig. 4 ). When the first Phe-tRNA Phe binds, the phenylalanyl side chain is accommodated in the catalytic pocket and both amino and carbonyl groups are appropriately positioned through hydrogen bonds with the side chains of E182 and Y178 (Step 1). The Y178 hydroxyl polarizes the incoming ester carbonyl of the first aa-tRNA and facilitates the nucleophilic attack by the S37 hydroxyl. S37 activation probably results from a concerted proton shuffling mechanism involving the two adjacent vicinal hydroxyls of the nucleotide A76 of the tRNA moiety [4] , as proposed for the ribosome at the peptidyl transferase centre [14] and the FemX aa-transferase of Weissella viridescens [15] . Then, the Y178 hydroxyl may help to stabilize the resulting phenylalanyl enzyme intermediate (Step 2). This is consistent with our structural data, indicating that Y178 is engaged in a polar contact with the carbonyl of Phe1 ( Fig. 2d ), and our previous finding showing that the Y178F substitution substantially impairs both enzymatic activity and the formation of the phenylalanyl enzyme intermediate [4] . Such a role for a Y hydroxyl has been described previously for prolyl oligopeptidase [16] and cocaine esterase [17] . Next, the second Phe-tRNA Phe binds (Step 3). The formation of the subsequent diphenylalanyl enzyme intermediate implies that the ammonium group of the phenylalanyl enzyme intermediate has to be deprotonated by a catalytic base to perform the nucleophilic attack on the incoming carbonyl of the second substrate. The nearby E182 may fulfill this role [13] , [18] , [19] . This residue is essential to the catalytic reaction and is involved in catalytic steps following amino-acyl formation [4] , [5] , [6] . Thus, the ammonium group of the first phenylalanine, deprotonated by the nearby carboxyl of E182, may attack the carbonyl group of the second Phe-tRNA Phe to generate a diphenylalanyl enzyme intermediate (Step 4). The carboxyl of E182 now in its protonated state may form electrostatic contacts with the two carbonyls of the dipeptide, similar to those we observed in the AlbC S37C-ZPK structure ( Fig. 2c ). The successive protonation states of E182 are supported further by pKa predictions made with the heuristic pKa calculation software PROPKA [20] (pKa values of 7.8 in free AlbC, 4.8 in the aminoacyl enzyme and 7.5 in AlbC S37C-ZPK). Thus, E182 and Y178 form hydrogen bonds with the dipeptide, precisely holding its backbone in the conformation required for cyclization. Y202 is then properly positioned to deprotonate the ammonium group of the second amino acid. Y202 participates in a hydrogen bond network, also involving N40 and H203, which are essential for the accurate positioning of catalytic residues. The substitution of either residue with alanine resulted in a dramatic impairment of enzymatic activity ( Supplementary Table 1 ) and phenylalanyl enzyme formation ( Supplementary Fig. 10 ), whereas the structural integrity of the variants was not affected ( Supplementary Fig. 7 ). Finally, Y202 would deprotonate the primary ammonium group to generate the nucleophile for attack at the enzyme ester bond (Step 5), leading to the formation of the cyclodipeptide product. 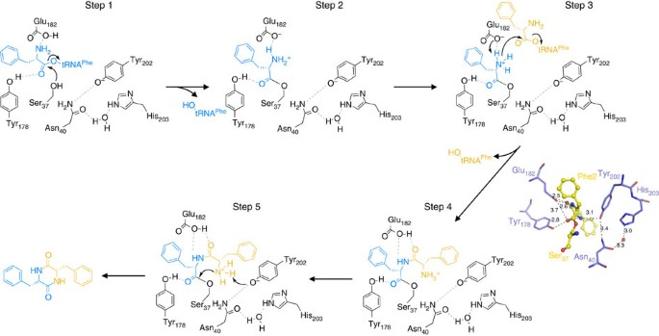Figure 4: Proposed mechanism for cyclodipeptide synthesis by CDPSs during which a covalent acyl- and subsequently dipeptidyl-AlbC are formed. The formation of cFF catalysed by AlbC is shown; the first and second incorporated phenylalanyl moieties of Phe-tRNAPheare highlighted in blue and yellow, respectively. Possible interactions are indicated by dashed lines and predicted distances are labelled. Step 4 is illustrated by the model of the diphenylalanyl enzyme intermediate in which residues involved in the catalysis are shown as blue sticks (seeSupplementary Fig. 6). The amino groups of Phe-tRNAs (Steps 1 and 3) are assumed to be in their NH2state, as described in the context of the ribosome32. The amino groups of the aminoacyl- (Steps 2 and 3) and dipeptidyl intermediates (Steps 4 and 5) are expected to be in their NH3+state33; these protonation states are supported by pKa values predicted with the heuristic pKa calculation software PROPKA20(10.4 and 11.2, respectively). Figure 4: Proposed mechanism for cyclodipeptide synthesis by CDPSs during which a covalent acyl- and subsequently dipeptidyl-AlbC are formed. The formation of cFF catalysed by AlbC is shown; the first and second incorporated phenylalanyl moieties of Phe-tRNA Phe are highlighted in blue and yellow, respectively. Possible interactions are indicated by dashed lines and predicted distances are labelled. Step 4 is illustrated by the model of the diphenylalanyl enzyme intermediate in which residues involved in the catalysis are shown as blue sticks (see Supplementary Fig. 6 ). The amino groups of Phe-tRNAs (Steps 1 and 3) are assumed to be in their NH 2 state, as described in the context of the ribosome [32] . The amino groups of the aminoacyl- (Steps 2 and 3) and dipeptidyl intermediates (Steps 4 and 5) are expected to be in their NH 3 + state [33] ; these protonation states are supported by pKa values predicted with the heuristic pKa calculation software PROPKA [20] (10.4 and 11.2, respectively). Full size image The AlbC-ZPK structure enables the identification of the two pockets P1 and P2 accommodating the aminoacyl moieties of the first and second aa-tRNA, respectively ( Fig. 2c,d ). We compared the residues lining P1 and P2 in all characterized CDPSs together with the cyclodipeptides that these enzymes produce ( Supplementary Table 2 and Supplementary Fig. 11 ). P1 has a hydrophobic character, in keeping with the accommodation of hydrophobic amino acids. Our structural data show that P2 is wider than P1, consistent with a somewhat relaxed specificity for the second aminoacyl moiety. In line with this idea, the amino acids lining P2 are poorly conserved ( Supplementary Table 2 ). This study, combining structural approaches and chemical biology experiments, elucidates the missing step in the mechanism of the recently discovered CDPSs—the formation of a dipeptidyl enzyme. Our work also identifies two different binding sites for the aminoacyl moieties of the two aa-tRNA substrates. We previously identified two different regions accommodating the tRNA moieties of the substrates [21] . Taken together, these data provide insight into the molecular basis of the interaction between CDPSs and their substrates. The first aa-tRNA binds to the enzyme through the accommodation of its aminoacyl moiety in the P1 pocket and the interaction of its tRNA moiety with basic residues located in the α4 helix that form a basic patch at the surface of the protein. When the acyl enzyme is formed, the second aa-tRNA binds with its aminoacyl moiety accommodated in the P2 pocket and its tRNA moiety interacting with residues of the α6–α7 loop. In both TyrRS and TrpRS, the loop equivalent to this α6–α7 loop is involved in tRNA binding [8] , [22] , [23] , [24] . CDPSs may have retained some characteristics of class-Ic aaRSs regarding their interaction with the tRNA moiety of the second substrate. Further studies describing precisely the tRNA-binding regions on CDPSs are still needed to clarify this issue. This study indicates that compared with class-Ic aaRSs, CDPSs have acquired both new active site residues and a new aminoacyl-binding site for a second aa-tRNA substrate. This is an important step forward in the understanding of CDPS specificity, and this knowledge may facilitate the engineering of these enzymes to produce a diversity of natural and unnatural cyclodipeptides. Purification of AlbC variants Plasmids encoding the AlbC variants S37C, Y202F and N40A were constructed previously [4] . The variant H203A was obtained via PCR mutagenesis with oligonucleotides described in Supplementary Table 3 of the plasmid pQE60-AlbC encoding C-terminal His 6 -tagged AlbC according to the QuikChange site-directed mutagenesis method (Stratagene). Sequences were verified by DNA sequencing. The C-terminal His 6 -tagged proteins were produced and purified as described previously [4] . Purified proteins were quantified by ultraviolet spectrophotometry. Protein molecular weights were verified by electrospray ionization MS (Esquire HCT ion trap mass spectrometer (Bruker Daltonik, GmbH)). The structural integrity of the variants was verified by far-ultraviolet circular dichroism spectroscopy (Jasco J-815 circular dichroism spectropolarimeter). Crystallization and structure determination A mixture of AlbC S37C (75 μM) and ZPCK (100 μM) was used for crystallization trials. Crystals were obtained by the sitting drop method at 4 °C (Mosquito robot, TTP Labtech), by mixing equal volumes of protein and a solution containing 10% (W/v) PEG8000, 50 mM KCl, 50 mM sodium cacodylate, pH 6.0 (condition E8 of the Natrix screen, Hampton Research). Cryoprotection was achieved by adding 25% (v/v) glycerol to the crystallization liquor. Diffraction data were collected at 100 K ( λ =0.984 Å) on the Proxima-1 beamline at the SOLEIL synchrotron equipped with a Pilatus detector. Diffraction images were analysed with X-ray Detector Software (XDS) [25] and the data were processed with programmes of the CCP4 package [26] . The final data set was at a resolution of 2.9 Å ( Table 1 ). The structure was solved by molecular replacement with PHASER [27] and the structure of AlbC [4] was used as a search model (PDB 3OQV ). Density for ZPCK connected to C37 was easily identified. The geometry restraints file for the ZPCK-modified cysteinyl residue was created with eLBOW and REEL [28] . The structure was refined through several cycles of manual rebuilding with COOT [29] and positional refinement with BUSTER (BUSTER version 2.10.0., Global Phasing Ltd, Cambridge, UK). A final round of refinement was performed with single group translation/libration/screw (TLS) parameters. The final model (free R =0.253, R =0.201) contained all AlbC residues, including the ZPCK-modified C37, with the exception of residues 1–9 at the amino terminus and residues 234–239 at the C terminus, as well as three water molecules. Refinement statistics are given in Table 1 . A model of the dipeptidyl enzyme was generated to facilitate interpretation by building a diphenylalanyl-modified serine residue from the refined ZPCK-modified cysteine coordinates and optimizing the geometry with eLBOW [28] . Acyl tRNA synthesis Production and purification of Escherichia coli tRNAs were performed as described previously [30] . tRNA Phe was expressed from pBSTNAV2/tRNA Phe (ref. 31 ) and tRNA LeuCAG from pBSTNAV2/tRNA LeuCAG (ref. 21 ). The concentration of aminoacylated tRNA was determined from plateau charging experiments [21] . Identification of the covalent peptidyl-enzyme species A total of 12 μM (2 equivalents) of Phe-tRNA Phe was mixed with 6 μM of AlbC (or variant) in 20 μl of the reaction buffer containing 50 mM HEPES-KOH pH 7.0 and 50 mM KCl. After 30 s of incubation, a 5-μl aliquot was removed and submitted to hydrolysis for further analysis by PMF: the samples were diluted up to 10 μl in 50 mM NH 4 AcO 2 , pH 8.0, and 1 μl of porcine trypsin (Promega) (400 ng μl −1 ) was added. Trypsinolysis was performed at 50 °C up to 10 min. Sample digests were then acidified by 1.25% trifluoroacetic acid (TFA) in water, desalted and concentrated by C18 ziptip and spotted with 4-HCCA matrix solution (10 mg ml −1 in 49.8/49.8/0.4: CH 3 CN/H 2 O/TFA: v/v/v) on a matrix-assisted laser desorption/ionization plate. The remaining reaction sample was analysed by LC–MS (ESI-ion trap Esquire HCT Bruker Daltonics) with a linear gradient of acetonitrile/water with 0.1% TFA (ProSwift RP-4H monolithic column from Thermo-Scientific). MS and MS/MS spectra were registered with a 4800 MALDI-TOF/TOF mass spectrometer (Applied Biosystems, Foster City, USA) in positive reflectron mode. Each MS spectrum was the result of 1,000 laser shots and trypsin autolysis fragments were used as internal standards for calibration. MS/MS analyses were performed under PSD (post-source decay) mode. Each MS/MS spectrum was the result of 10,000 shots. The sequence of the trypsin fragments was identified with Data Explorer processing software (Version 4.9, Applied Biosystems) to assign the potential chemical modifications of the serine or cysteine residues. AlbC S37C-ZPK characterization AlbC S37C (0.04 μg μl −1 ) was incubated with 100 equivalents of ZPCK in Tris–HCl 100 mM, pH 8 for 3 h. The sample was loaded onto a Ni-NTA agarose resin (Qiagen) to wash out the excess ZPCK. The resin was washed with a large excess of 50 mM HEPES-KCl, 50 mM KCl buffer. A 5-μl aliquot of resin was removed, diluted up to 10 μl in 50 mM NH 4 AcO 2 , pH 8.0, and submitted to trypsin digestion for PMF as described for the identification of the peptidyl enzyme intermediate. Cyclodipeptide-synthesizing activity assay The CDPS activity of AlbC and AlbC variants was measured with an end point assay, as performed previously [21] . Activity was determined in a coupled assay containing aaRSs to generate in situ the aa-tRNA substrates. The assay was performed in a buffer containing 50 mM HEPES-KOH, pH 7.5, 50 mM KCl, 15 mM MgCl 2 , 0.1 mM EDTA, 2 mM ATP, 10 mM β-mercaptoethanol), with 50 μM Phe and Leu, 1 μM PheRS and LeuRS, 150 nM AlbC or 1.5 μM AlbC variant, 0.75 μM Phe-tRNA Phe and 0.66 μM Leu-tRNA LeuCAG . The reaction was carried out at 30 °C with a preincubation of 15 min with the aaRSs for the synthesis of aa-tRNAs before the addition of AlbC or AlbC variant. The enzymatic reaction was initiated by the addition of AlbC or AlbC variant. The reaction was stopped after 21 min by acidification with 2% TFA, and mixed with known concentrations of stable isotope internal standards ( 13 C 9 , 15 N-labelled cFF and cFL solutions), before cFF and cFL quantification by LC–MS as described previously [7] . How to cite this article: Moutiez, M. et al. Unravelling the mechanism of non-ribosomal peptide synthesis by cyclodipeptide synthases. Nat. Commun. 5:5141 doi: 10.1038/ncomms6141 (2014). Accession codes: The atomic coordinates and the structure factors have been deposited with the accession code 4Q24.